Orphan receptor IL-17RD tunes IL-17A signalling and is required for neutrophilia Interleukin-17A, the prototypical member of the interleukin-17 cytokine family, coordinates local tissue inflammation by recruiting neutrophils to sites of infection. Dysregulation of interleukin-17 signalling has been linked to the pathogenesis of inflammatory diseases and autoimmunity. The interleukin-17 receptor family members (A–E) have a broad range of functional effects in immune signalling yet no known role has been described for the remaining orphan receptor, interleukin-17 receptor D, in regulating interleukin-17A-induced signalling pathways. Here we demonstrate that interleukin-17 receptor D can differentially regulate the various pathways employed by interleukin-17A. Neutrophil recruitment, in response to in vivo administration of interleukin-17A, is abolished in interleukin-17 receptor D-deficient mice, correlating with reduced interleukin-17A-induced activation of p38 mitogen-activated protein kinase and expression of the neutrophil chemokine MIP-2. In contrast, interleukin-17 receptor D deficiency results in enhanced interleukin-17A-induced activation of nuclear factor-kappa B and interleukin-6 and keratinocyte chemoattractant expression. Interleukin-17 receptor D disrupts the interaction of Act1 and TRAF6 causing differential regulation of nuclear factor-kappa B and p38 mitogen-activated protein kinase signalling pathways. Pro-inflammatory cytokines of the interleukin-17 (IL-17) family are secreted by cells of the activated immune system, including T H 17 cells, γδ-T cells and natural killer cells, and contribute to host defence against extracellular pathogens [1] . IL-17 signalling pathways are also implicated in the pathogenesis of auto-immune and inflammatory diseases, and IL-17 is found in increased concentrations in psoriasis, rheumatoid arthritis, inflammatory bowel disease and the lungs of patients with allergic asthma [2] , [3] , [4] , [5] . The IL-17 cytokine family consists of six ligands (IL-17A-F), which signal through five receptors (IL-17RA-E). IL-17 receptors are widely expressed bestowing the cytokines with broad effector functions [6] , [7] . To date, IL-17RA and IL-17RC have been the best-characterized members of the IL-17 receptor family, and IL-17RA can form heterodimers with IL-17RC in initiating immune responses to extracellular pathogens [8] . IL-17A and IL-17F can form homodimers or heterodimers and IL-17RA- and IL-17RC-deficient mice show impaired responsiveness to both ligands [9] , [10] . IL-17RA binds to IL-17A with a higher affinity than IL-17F in humans, whereas the converse is true of IL-17RC [11] . Murine IL-17RA can bind both IL-17A and IL-17F but murine IL-17RC can only bind IL-17F. Recent findings have revealed a new role for IL-17RE in intestinal immunity in response to bacterial infection, with IL-17RE forming a receptor complex with IL-17RA to bind IL-17C [12] , [13] , [14] . IL-17A coordinates tissue inflammation and mobilizes neutrophils by stimulating the production of cytokines and chemokines, including IL-6, keratinocyte chemoattractant (KC) and macrophage inflammatory protein-2 (MIP-2) in mice, and IL-8 and growth-regulated oncogene family members in humans [15] , [16] , [17] , [18] . IL-17RA regulates gene expression by activating nuclear factor-kappa B (NF-κB) and mitogen-activated protein kinase (MAPK) pathways [18] . Members of the IL-17 receptor family share an intracellular Sef/IL-17R (SEFIR) domain that is important for triggering downstream signalling [19] . Stimulation of IL-17RA leads to an association with the adaptor Act1, via SEFIR–SEFIR interactions, followed by recruitment and polyubiquitination of TRAF6, thus initiating downstream activation of NF-κB and MAPKs [20] , [21] . Recent findings have also detailed a messenger RNA (mRNA)-stability pathway bifurcating downstream of Act1 that is independent of TRAF6 (ref. 22 ). Although recent studies have delineated important immunomodulatory roles for the various IL-17R members, IL-17 receptor D (IL-17RD) remains an orphan receptor with no reported physiological role in IL-17 signalling, apart from a study in which overexpression of IL-17RD was shown to co-operate with IL-17RA [23] . IL-17RD was originally termed similar expression to fgf (Sef) due its coexpression with fgf genes in zebrafish embryo development [24] . Here, we describe for the first time an important physiological role for IL-17RD in IL-17 signalling. IL-17RD negatively regulates IL-17A-induced activation of NF-κB and the expression of pro-inflammatory genes such as IL-6 . IL-17RD coordinates these regulatory effects by negatively regulating Act1/TRAF6 binding and disrupting the IL-17RA/Act1/TRAF6 signalling axis. However, conversely IL-17RD promotes IL-17A-induced activation of p38 MAPK and induction of MIP-2. In vivo , the loss of IL-17A-induced MIP-2 expression in IL-17RD-deficient mice is associated with diminished IL-17A-induced neutrophil infiltration in the lungs and the peritoneum, whereas exogenous MIP-2 delivery restores neutrophilia in these mice. From these findings it is evident that IL-17RD differentially regulates IL-17A-induced NF-κB and MAPK signalling pathways, and is an important mediator in facilitating IL-17A-induced neutrophilia. IL-17RD knockdown increases responsiveness to IL-17A To elucidate the role of IL-17RD in IL-17A signalling, we first assessed the effects of IL-17RD knockdown on IL-17A-induced activation of NF-κB. HeLa cells were co-transfected with an NF-κB-regulated luciferase reporter plasmid and IL-17RD-specific small interfering RNA (siRNA) or a scrambled control siRNA. The IL-17RD-specific siRNA strongly suppressed IL-17RD expression whereas the control siRNA was without effect ( Fig. 1a ). Knockdown of IL-17RD augmented the ability of human IL-17A to induce the expression of NF-κB-regulated luciferase ( Fig. 1a ). The control siRNA was without effect confirming the specificity of the effects of IL-17RD siRNA. Additionally, IL-17A-induced expression of the NF-κB-responsive gene IL-6 was enhanced in IL-17RD-knockdown cells ( Fig. 1b ), consistent with an inhibitory role for IL-17RD in regulating IL-17A-induced activation of NF-κB. This was further confirmed by overexpressed IL-17RD inhibiting IL-17A-induced activation of NF-κB activation in HeLa cells ( Fig. 1c ). 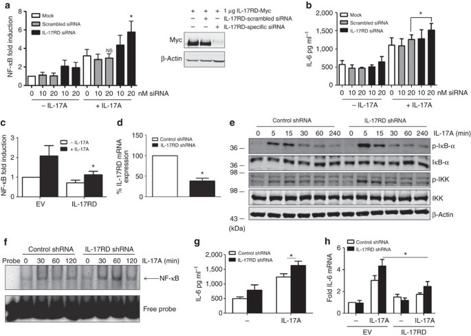Figure 1: Knockdown of human IL-17RD enhances IL-17A-induced signalling. (a) Assay of NF-κB reporter activity in HeLa cells transfected with IL-17RD-specific siRNA or scrambled siRNA (10, 20 nM). Forty-eight hours post transfection cells were treated with IL-17A (100 ng ml−1) for 8 h. The efficiency of silencing was evaluated by immunoblotting (right panel). (b) Cell supernatants were assayed for IL-6 levels by sandwich ELISA. (c) NF-κB reporter assay in HeLa cells transfected overnight with IL-17RD (100 ng) or empty vector pcDNA3.1 (EV). Transfected cells were then treated with IL-17A (100 ng ml−1) for 8 h. (d) Knockdown of IL-17RD mRNA in U373 cells stably transduced with control shRNA or specific IL-17RD shRNA. U373 cells stably transduced with control shRNA or IL-17RD-specific shRNA were treated with IL-17RA (100 ng ml−1) as indicated. Cells lysates were subjected to immunoblotting with indicated antibodies (e) or nuclear extracts were assayed for NF-κB/DNA binding by electrophoretic mobility shift assay (f) or supernatants were analysed for IL-6 production using sandwich ELISA (g). (h) U373 cells stably transduced with control shRNA or IL-17RD-specific shRNA were transfected with EV or IL-17RD (1 μg). Cells were then treated with IL-17A (100 ng ml−1) for 24 h and IL-6 mRNA levels were evaluated by quantitative PCR (qPCR). Data are representative of three independent experiments (e,f) or represent mean±s.e.m. of three independent experiments (a–d,g–h) with triplicate determinants (a–c,g–h). NS, nonsignificant; *P<0.05 (Student'sttest). Figure 1: Knockdown of human IL-17RD enhances IL-17A-induced signalling. ( a ) Assay of NF-κB reporter activity in HeLa cells transfected with IL-17RD-specific siRNA or scrambled siRNA (10, 20 nM). Forty-eight hours post transfection cells were treated with IL-17A (100 ng ml −1 ) for 8 h. The efficiency of silencing was evaluated by immunoblotting (right panel). ( b ) Cell supernatants were assayed for IL-6 levels by sandwich ELISA. ( c ) NF-κB reporter assay in HeLa cells transfected overnight with IL-17RD (100 ng) or empty vector pcDNA3.1 (EV). Transfected cells were then treated with IL-17A (100 ng ml −1 ) for 8 h. ( d ) Knockdown of IL-17RD mRNA in U373 cells stably transduced with control shRNA or specific IL-17RD shRNA. U373 cells stably transduced with control shRNA or IL-17RD-specific shRNA were treated with IL-17RA (100 ng ml −1 ) as indicated. Cells lysates were subjected to immunoblotting with indicated antibodies ( e ) or nuclear extracts were assayed for NF-κB/DNA binding by electrophoretic mobility shift assay ( f ) or supernatants were analysed for IL-6 production using sandwich ELISA ( g ). ( h ) U373 cells stably transduced with control shRNA or IL-17RD-specific shRNA were transfected with EV or IL-17RD (1 μg). Cells were then treated with IL-17A (100 ng ml −1 ) for 24 h and IL-6 mRNA levels were evaluated by quantitative PCR (qPCR). Data are representative of three independent experiments ( e , f ) or represent mean±s.e.m. of three independent experiments ( a–d , g–h ) with triplicate determinants ( a–c , g–h ). NS, nonsignificant; * P <0.05 (Student's t test). Full size image To further validate these effects, we established U373 cell lines transduced with lentivirus to stably express IL-17RD-specific short-hairpin RNA (shRNA) or control shRNA. Knockdown efficiency was regularly checked in these U373-shRNA stable cell lines and 40–60% knockdown of Il17rd mRNA was consistently achieved compared with the control-shRNA ( Fig. 1d ). The knockdown of IL-17RD in these cells resulted in augmented IL-17A-induced phosphorylation of IκB and upstream IKKs ( Fig. 1e ) and this was associated with enhanced NF-κB–DNA binding ( Fig. 1f ). Again, knockdown of IL-17RD in this model resulted in an enhancement of IL-17A-induced expression of IL-6 ( Fig. 1g ). To further validate that augmented IL-6 production in IL-17RD-knockdown cells is directly attributable to diminished expression of IL-17RD, we demonstrated that the expression of exogenous IL-17RD strongly suppressed IL-17A induction of IL-6 in cells stably expressing IL-17RD shRNA ( Fig. 1h ). IL-17RD differentially regulates IL-17A-responsive genes The above knockdown studies suggested IL-17RD to be a negative regulator of IL-17A signalling. To confirm the physiological relevance of such a role, it was necessary to generate IL-17RD-deficient mice and this was achieved by gene-trap technology. The gene that encodes murine IL-17RD consists of 13 exons. The targeting vector disrupted the Il17rd gene between the first and second exons with a β-geomycin-resistance gene cassette ( Supplementary Fig. S1a ). Il17rd −/− pups were born in an expected Mendelian ratio and showed no obvious phenotypic abnormalities and this is consistent with previously generated IL-17RD-deficient mice [25] . As expected, Il17rd mRNA expression is abolished in Il17rd −/− mice and replaced by β-Geo expression ( Supplementary Fig. S1b ). Quantitative PCR was used to confirm disruption of the gene encoding IL-17RD in Il17rd −/− murine embryonic fibroblasts (MEFs) ( Supplementary Fig. S1c ). Il17rd −/− MEFs were used to assess a potential regulatory role for IL-17RD by measuring IL-6 expression in response to principal IL-17RA cytokines, IL-17A and IL-17F ( Fig. 2a ). IL-17A was the more efficacious inducer of IL-6 expression from MEFs from wild-type mice and its efficacy was greatly enhanced in Il17rd −/− MEFS. A more detailed characterization of the regulatory effects of IL-17RD on IL-17A signalling was then performed. This initially involved an assessment of the effects of IL-17RD deficiency on the expression of a number of IL-17A-responsive genes in MEFs. Similar to IL-6, loss of IL-17RD resulted in significantly enhanced KC expression in response to IL-17A ( Fig. 2b ). In contrast IL-17A-induced expression of the chemokine MIP-2 was diminished in Il17rd −/− MEFs, indicating that IL-17RD can differentially regulate the expression of IL-17A-responsive genes. This was independent of cell type as primary bone marrow-derived macrophages (BMDMs) from Il17rd −/− mice also displayed enhanced expression of IL-6 and KC but reduced expression of MIP-2 in response to IL-17A ( Fig. 2c ). The differential effects of loss of IL-17RD on KC and MIP-2 expression are also relevant to human cells as U373 cells, stably expressing IL-17RD shRNA, similarly showed diminished production of human MIP-2 but increased IL-8 gene expression upon administration of human IL-17A ( Fig. 2d ). We further validated the findings in human primary cells. Thus, peripheral blood mononuclear cells (PBMCs) were isolated from blood, obtained from healthy volunteers, and transfected with IL-17RD-specific and scrambled siRNAs to silence IL-17RD gene expression ( Fig. 2e ). Knockdown of IL-17RD in PBMCs resulted in diminished human MIP-2 production and an increase in IL-8 protein expression in response to IL-17A ( Fig. 2e ). These studies indicate that IL-17RD exerts differential effects on the expression of IL-17-responsive genes with the loss of IL-17RD leading to augmented induction of IL-6 and KC (IL-8 in human cells) but suppressed expression of MIP-2. 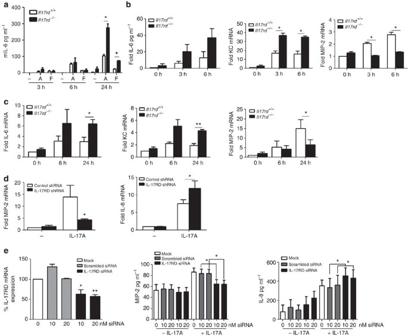Figure 2: IL-17RD differentially regulates expression of IL-17A-responsive genes. (a) Primary MEFs fromIl17rd+/+andIl17rd−/−mice were treated with IL-17 ligands (100 ng ml−1) as indicated and IL-6 production was assayed by ELISA. Primary MEFs (b) and BMDMs (c) fromIl17rd+/+andIl17rd−/−mice were incubated with IL-17A (100 ng ml−1) as indicated. IL-6, KC and MIP-2 mRNA levels were evaluated by qPCR. (d) U373 cells, stably transduced with control shRNA or IL-17RD-specific shRNA, were treated with IL-17A (100 ng ml−1) for 24 h. Human MIP-2 and IL-8 mRNA levels were evaluated by qPCR. (e) Primary human PBMCs were transfected with IL-17RD-specific or scrambled siRNA for 48 h and treated with human IL-17A for 24 h. The efficiency of gene silencing was measured by qPCR. Human MIP-2 and IL-8 protein levels were measured by ELISA. Data represent mean±s.e.m. of three independent experiments (a–e) with triplicate determinants. *P<0.05; **P<0.01 (Student'sttest). Figure 2: IL-17RD differentially regulates expression of IL-17A-responsive genes. ( a ) Primary MEFs from Il17rd +/+ and Il17rd −/− mice were treated with IL-17 ligands (100 ng ml −1 ) as indicated and IL-6 production was assayed by ELISA. Primary MEFs ( b ) and BMDMs ( c ) from Il17rd +/+ and Il17rd −/− mice were incubated with IL-17A (100 ng ml −1 ) as indicated. IL-6, KC and MIP-2 mRNA levels were evaluated by qPCR. ( d ) U373 cells, stably transduced with control shRNA or IL-17RD-specific shRNA, were treated with IL-17A (100 ng ml −1 ) for 24 h. Human MIP-2 and IL-8 mRNA levels were evaluated by qPCR. ( e ) Primary human PBMCs were transfected with IL-17RD-specific or scrambled siRNA for 48 h and treated with human IL-17A for 24 h. The efficiency of gene silencing was measured by qPCR. Human MIP-2 and IL-8 protein levels were measured by ELISA. Data represent mean±s.e.m. of three independent experiments ( a–e ) with triplicate determinants. * P <0.05; ** P <0.01 (Student's t test). Full size image IL-17RD mediates neutrophil infiltration to the peritoneum Given the above differential effects of IL-17RD on IL-17A-responsive genes, we next probed the physiological relevance of these effects by evaluating IL-17A-mediated neutrophilia in both Il17rd +/+ and Il17rd −/− mice. Mice were treated with recombinant IL-17A via intraperitoneal injection, killed 3 h post injection and peritoneal cells were collected from lavage. Flow cytometric analysis was subsequently performed on the peritoneal exudate cells (PECs) to quantitate the neutrophil population ( Fig. 3a ). The administration of IL-17A to wild-type mice induced marked neutrophil infiltration into the peritoneum but this was dramatically reduced in Il17rd −/− mice. The greatly diminished neutrophil infiltration in Il17rd −/− mice was observed at various times post IL-17A administration ( Fig. 3b ). The critical mediatory role for IL-17RD in facilitating neutrophil infiltration was selective for IL-17A signalling as neutrophil infiltration trigged by the bacterial chemoattractant peptide formyl–Met–Leu–Phe was unaffected by loss of IL-17RD ( Fig. 3c ). We next measured the expression of IL-6, KC and MIP-2 in PECs isolated from the above treated mice. The in vivo administration of IL-17A increased the mRNA levels of all three cytokines in PECs from wild-type mice and in keeping with the earlier cell-based models, the induction of IL-6 and KC was further enhanced whereas MIP-2 expression was greatly diminished in PECs from similarly treated Il17rd −/− mice ( Fig. 3d ). These findings were further corroborated by measuring KC and MIP-2 protein levels in lavage fluid from IL-17-treated mice. Again administration of IL-17A to wild-type mice caused increased lavage levels of KC and MIP2, with KC being further enhanced and MIP-2 diminished in similarly treated Il17rd −/− mice ( Fig. 3e ). Given that IL-17A-induced expression of MIP-2 is greatly suppressed in Il17rd −/− mice, coupled to the strong chemoattractant activity of MIP-2 towards neutrophils, we investigated whether administration of exogenous MIP-2 could overcome the deficiency in IL-17A-induced neutrophilia that we observed in Il17rd −/− mice. We again treated mice with IL-17A by intraperitoneal injection, which was followed by intraperitoneal injection of recombinant MIP-2 one hour later in order to evaluate whether MIP-2 deficiency provided an underlying basis to the phenotypic changes on neutrophilia in Il17rd −/− mice. As before, the administration of IL-17A to wild-type mice promoted strong neutrophilia and this was not further enhanced by coadministration of MIP-2, indicating that the latter is not a limiting factor in wild-type mice ( Fig. 3f ). However, exogenous MIP-2 significantly enhanced neutrophilia in IL-17A-treated Il17rd −/− mice consistent with our hypothesis that deficiency in MIP-2 expression in IL-17RD-deficient mice may be an important limiting factor underlying reduced neutrophilia in these animals ( Fig. 3f ). It is interesting to note that the enhanced KC expression in Il17rd −/− mice failed to compensate for the reduced levels of MIP-2. However, a previous study indicated MIP-2 to be a more potent neutrophil chemoattractant than KC [26] . Our findings are consistent with this role for MIP-2 being the chief chemoattractant of neutrophils in vivo , as the diminished IL-17A-induced neutrophil infiltration in Il17rd −/− mice was associated with loss of MIP-2 expression. 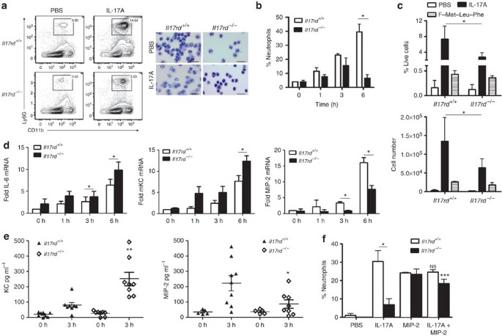Figure 3: IL-17RD deficiency impairs neutrophil recruitment to the peritoneum. (a,b) IL-17A (0.5 μg per mouse) or PBS was administered by intraperitoneal injection intoIl17rd+/+andIl17rd−/−mice. (a) Representative flow cytometry plots of neutrophil infiltration, using CD11b and Ly6G expression as markers, 3 h after PBS or IL-17A injection (left panel). Wright's staining of infiltrate fromIl17rd+/+andIl17rd−/−mice (right panel). Scale bar, 10 μm. (b) Percentages of neutrophils in peritoneal lavages from mice treated with IL-17A as indicated. (c) IL-17A (0.5 μg per mouse), formyl-Met–Leu–Phe (1 μg per mouse) or PBS was injected into the peritoneum ofIl17rd+/+andIl17rd−/−mice. Data indicate percentage (upper panel) and absolute numbers (lower panel) of neutrophils. (d)Il17rd+/+andIl17rd−/−mice were injected intraperitoneal with IL-17A (0.5 μg per mouse). Peritoneal cells were collected from mice treated with IL-17A as indicated. IL-6, KC and MIP-2 mRNA levels were evaluated by quantitative PCR. (e) ELISA of MIP-2 and KC levels from peritoneal lavages from mice treated with IL-17A as indicated. (f) Percentages of neutrophils in peritoneal lavages from mice treated with IL-17A or PBS for 1 h before intraperitoneal injection of murine recombinant MIP-2 (30 ng) for 2 h. Results are mean±s.e.m. (n=4–7 mice per group) and data are representative of three individual experiments (totaln=12–21) (a–c), represent mean±s.e.m. of three independent experiments (totaln=8–9) (d–e) or are mean±s.e.m. (totaln=4–9) (f). *P<0.05; **P<0.01; ***P<0.001 (Student'sttest). NS, nonsignificant. Figure 3: IL-17RD deficiency impairs neutrophil recruitment to the peritoneum. ( a , b ) IL-17A (0.5 μg per mouse) or PBS was administered by intraperitoneal injection into Il17rd +/+ and Il17rd −/− mice. ( a ) Representative flow cytometry plots of neutrophil infiltration, using CD11b and Ly6G expression as markers, 3 h after PBS or IL-17A injection (left panel). Wright's staining of infiltrate from Il17rd +/+ and Il17rd −/− mice (right panel). Scale bar, 10 μm. ( b ) Percentages of neutrophils in peritoneal lavages from mice treated with IL-17A as indicated. ( c ) IL-17A (0.5 μg per mouse), formyl-Met–Leu–Phe (1 μg per mouse) or PBS was injected into the peritoneum of Il17rd +/+ and Il17rd −/− mice. Data indicate percentage (upper panel) and absolute numbers (lower panel) of neutrophils. ( d ) Il17rd +/+ and Il17rd −/− mice were injected intraperitoneal with IL-17A (0.5 μg per mouse). Peritoneal cells were collected from mice treated with IL-17A as indicated. IL-6, KC and MIP-2 mRNA levels were evaluated by quantitative PCR. ( e ) ELISA of MIP-2 and KC levels from peritoneal lavages from mice treated with IL-17A as indicated. ( f ) Percentages of neutrophils in peritoneal lavages from mice treated with IL-17A or PBS for 1 h before intraperitoneal injection of murine recombinant MIP-2 (30 ng) for 2 h. Results are mean±s.e.m. ( n =4–7 mice per group) and data are representative of three individual experiments (total n =12–21) ( a–c ), represent mean±s.e.m. of three independent experiments (total n =8–9) ( d–e ) or are mean±s.e.m. (total n =4–9) ( f ). * P <0.05; ** P <0.01; *** P <0.001 (Student's t test). NS, nonsignificant. Full size image IL-17RD mediates IL-17A-induced pulmonary neutrophilia The key role of IL-17RD in mediating neutrophil infiltration into the peritoneum in response to IL-17A prompted us to examine a more general role for IL-17RD in mediating tissue neutrophilia. To investigate this, mice were challenged with IL-17A via intranasal injection to elicit pulmonary neutrophilia. Mice were killed after 24 h and cells in the bronchoalveloar lavage (BAL) fluid were analysed ( Fig. 4a ). Consistent with findings from intraperitoneal injection, Il17rd −/− mice had significantly less ( P <0.038, Student's t test) lung-infiltrating neutrophils, in response to IL-17A administration, in the BAL fluid relative to wild-type animals ( Fig. 4a ). There was no difference in lymphocyte and monocyte numbers in BAL fluid between Il17rd +/+ and Il17rd −/− mice, demonstrating a specific effect of IL-17RD on neutrophilia. Furthermore, histological analysis of lung tissue showed a significant decrease in neutrophil infiltration in Il17rd −/− mice compared with Il17rd +/+ mice ( Fig. 4b ). 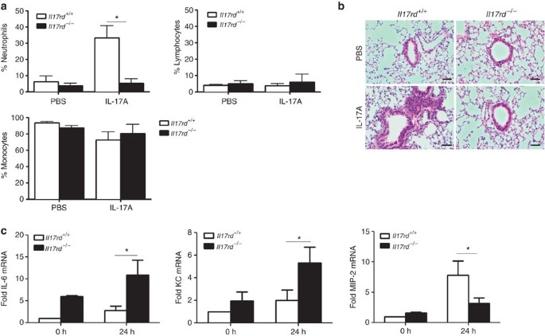Figure 4: IL-17RD regulates IL-17A-induced neutrophil infiltration in lung tissue. (a,b) IL-17A (0.5 μg per mouse) was introduced intranasally intoIl17rd+/+andIl17rd−/−mice. (a) Differential cell count data from cytospin slides depicting percentages of neutrophils, lymphocytes and monocytes in BAL at 4 h after IL-17A treatment. (b) Representative images of hematoxylin and eosin stained slides from lungs taken fromIl17rd+/+andIl17rd−/−mice after IL-17A treatment. Scale bar, 50 μm. (c) IL-17A (0.5 μg) was introduced intranasally for 24 h and lung tissue was retained to measure mRNA levels of IL-6, KC and MIP-2 by quantitative PCR (qPCR). Results are mean±s.e.m. (n=3–4 mice per group) and data are representative of three independent experiments (totaln=9–12) (a,b) or are mean±s.e.m. (n=4–6 mice per group) (c). *P<0.05 (Student'sttest). Figure 4: IL-17RD regulates IL-17A-induced neutrophil infiltration in lung tissue. ( a , b ) IL-17A (0.5 μg per mouse) was introduced intranasally into Il17rd +/+ and Il17rd −/− mice. ( a ) Differential cell count data from cytospin slides depicting percentages of neutrophils, lymphocytes and monocytes in BAL at 4 h after IL-17A treatment. ( b ) Representative images of hematoxylin and eosin stained slides from lungs taken from Il17rd +/+ and Il17rd −/− mice after IL-17A treatment. Scale bar, 50 μm. ( c ) IL-17A (0.5 μg) was introduced intranasally for 24 h and lung tissue was retained to measure mRNA levels of IL-6, KC and MIP-2 by quantitative PCR (qPCR). Results are mean±s.e.m. ( n =3–4 mice per group) and data are representative of three independent experiments (total n =9–12) ( a , b ) or are mean±s.e.m. ( n =4–6 mice per group) ( c ). * P <0.05 (Student's t test). Full size image IL-17A-induced expression of IL-6, KC and MIP-2 was also measured in lung tissue from the above mice by quantitative PCR ( Fig. 4c ). IL-17A-induced expression of KC and IL-6 levels was further augmented in lung tissue from Il17rd −/− mice relative to Il17rd +/+ mice, whereas IL-17A-induced MIP-2 expression was greatly reduced in lung samples from Il17rd −/− mice. This is consistent with the observed absence of neutrophilia in the lung and reaffirms a critical role for IL-17RD as a mediator of neutrophilia. IL-17RD differentially regulates NF-κB and p38 MAPK To understand the mechanism by which IL-17RD can differentially regulate the expression of IL-17A-responsive genes, we characterized the role of IL-17RD in IL-17 signalling pathways. IL-17A-induced signalling diverges at Act1 into TRAF6-dependent and -independent pathways. In the TRAF6-independent pathway, Act1 recruits TRAF2 and TRAF5, which in turn dissociate splicing-regulatory factor 2 from the 3′-untranslated region (3′UTR) of mRNAs, such as those encoding KC, thus promoting stability of the mRNA [22] . However, IL-17RD appears to lack a role in this arm of the IL-17A signalling pathway as KC and MIP-2 mRNA show similar stability profiles in MEFs from Il17rd +/+ and Il17rd −/− embryos ( Supplementary Fig. S2a ). In addition overexpression of IL-17RD failed to affect the Act1 induction of a luciferase reporter gene with 3′-UTRs from various IL-17-responsive genes ( Supplementary Fig. S2b ). In the TRAF6-dependent pathway arm of the IL-17A pathway, Act1 recruits TRAF6, promoting ubiquitination of the latter and activation of NF-κB and MAPKs. In a further effort to understand the mechanism(s) by which IL-17RD can exert differential regulatory effects on the expression of IL-17A-responsive genes, we characterized the ability of IL-17A to activate the NF-κB and MAPK pathways in primary macrophages from Il17rd +/+ and Il17rd −/− mice. Loss of IL-17RD results in increased IL-17A-induced phosphorylation of IκB ( Fig. 5a ). In relation to the MAPK pathways, the most notable IL-17RD-mediated response was marked reduction in p38 MAPK phosphorylation. These differential effects of IL-17RD on IL-17A-induced activation of NF-κB and p38 MAPK were also observed in Il17rd −/− MEFs ( Supplementary Fig. S3 ). 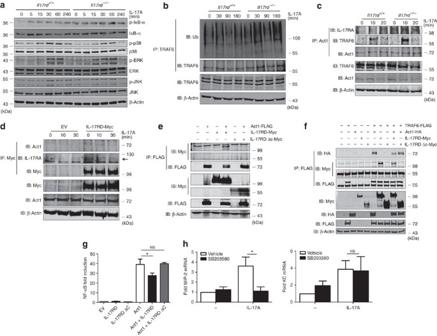Figure 5: IL-17RD targets Act1 and differentially regulates NF-κB and p38 MAPK. (a) Primary BMDMs fromIl17rd+/+andIl17rd−/−mice were stimulated with IL-17A (100 ng ml−1) as indicated. Cell lysates were subjected to immunoblotting with indicated antibodies. (b) Primary MEFs fromIl17rd+/+andIl17rd−/−embryos were stimulated with IL-17A (100 ng ml−1) as indicated. Cell lysates were immunoprecipitated with anti-TRAF6 and treated with SDS followed by immunoblotting with indicated antibodies. (c) Primary MEFs fromIl17rd+/+andIl17rd−/−embryos were stimulated with IL-17A (100 ng ml−1) as indicated. Cell lysates were immunoprecipitated with anti-Act1 followed by immunoblotting with indicated antibodies. (d) HeLa cells were transfected for 24 h with IL-17RD-Myc or EV (5 μg) in 90 mm petri dishes. Cells were then treated with IL-17A (100 ng ml−1) as indicated. Lysates were immunoprecipitated with anti-Myc followed by immunoblotting with indicated antibodies. (e) HEK293 cells were transfected for 24 h with Act1-FLAG, IL-17RD-Myc or IL-17RD ΔC-Myc (1 μg). Lysates were immunoprecipitated with anti-FLAG, followed by immunoblotting with indicated antibodies. (f) HEK293 cells were transfected for 24 h with Act1-HA, TRAF6-FLAG and IL-17RD-Myc or IL-17RD ΔC-Myc (1 μg). Lysates were immunoprecipitated with anti-FLAG, followed by immunoblotting with indicated antibodies. (g) NF-κB reporter assay in HEK293 cells transfected overnight with Act1 (50 ng) with IL-17RD or IL-17RD ΔC (50 ng). (h) Primary BMDMs fromIl17rd+/+andIl17rd−/−mice were pre-treated for 45 min with SB203580 (10 μM) and then stimulated with IL-17A (100 ng ml−1) for 3 h. MIP-2 and KC mRNA levels were evaluated by qPCR. Data are representative of three independent experiments (a–f) or represent mean±s.e.m. of three independent experiments (g,h). *P<0.05 (Student'sttest). NS, nonsignificant. Figure 5: IL-17RD targets Act1 and differentially regulates NF-κB and p38 MAPK. ( a ) Primary BMDMs from Il17rd +/+ and Il17rd −/− mice were stimulated with IL-17A (100 ng ml −1 ) as indicated. Cell lysates were subjected to immunoblotting with indicated antibodies. ( b ) Primary MEFs from Il17rd +/+ and Il17rd −/− embryos were stimulated with IL-17A (100 ng ml −1 ) as indicated. Cell lysates were immunoprecipitated with anti-TRAF6 and treated with SDS followed by immunoblotting with indicated antibodies. ( c ) Primary MEFs from Il17rd +/+ and Il17rd −/− embryos were stimulated with IL-17A (100 ng ml −1 ) as indicated. Cell lysates were immunoprecipitated with anti-Act1 followed by immunoblotting with indicated antibodies. ( d ) HeLa cells were transfected for 24 h with IL-17RD-Myc or EV (5 μg) in 90 mm petri dishes. Cells were then treated with IL-17A (100 ng ml −1 ) as indicated. Lysates were immunoprecipitated with anti-Myc followed by immunoblotting with indicated antibodies. ( e ) HEK293 cells were transfected for 24 h with Act1-FLAG, IL-17RD-Myc or IL-17RD ΔC-Myc (1 μg). Lysates were immunoprecipitated with anti-FLAG, followed by immunoblotting with indicated antibodies. ( f ) HEK293 cells were transfected for 24 h with Act1-HA, TRAF6-FLAG and IL-17RD-Myc or IL-17RD ΔC-Myc (1 μg). Lysates were immunoprecipitated with anti-FLAG, followed by immunoblotting with indicated antibodies. ( g ) NF-κB reporter assay in HEK293 cells transfected overnight with Act1 (50 ng) with IL-17RD or IL-17RD ΔC (50 ng). ( h ) Primary BMDMs from Il17rd +/+ and Il17rd −/− mice were pre-treated for 45 min with SB203580 (10 μM) and then stimulated with IL-17A (100 ng ml −1 ) for 3 h. MIP-2 and KC mRNA levels were evaluated by qPCR. Data are representative of three independent experiments ( a–f ) or represent mean±s.e.m. of three independent experiments ( g , h ). * P <0.05 (Student's t test). NS, nonsignificant. Full size image As IL-17RD −/− cells showed enhanced NF-κB activation in response to IL-17A, compared with their wild-type counterparts, we examined the effect of the loss of IL-17RD on the ubiquitination status of TRAF6. Polyubiquitination of TRAF6 was enhanced in IL-17RD-deficient cells ( Fig. 5b ), which is consistent with the increased activation of NF-κB. As IL-17RA employs Act1 to promote the polyubiquitination of TRAF6, we next investigated the potential of IL-17RD to regulate the interaction of Act1 with IL-17RA and TRAF6. We demonstrate that IL-17A-induced interaction of Act1 with both TRAF6 and IL-17RA is further enhanced in IL-17RD-deficient MEFs, consistent with a role for IL-17RD in inhibiting this arm of the pathway ( Fig. 5c ). The increased interaction of Act1 with TRAF6 correlates with the increased polyubiquitination of TRAF6 and activation of NF-κB in response to IL-17A in IL-17RD-deficient cells. These data suggest that IL-17RD may act as a natural 'brake' for IL-17A signalling by inhibiting the interaction of Act1 with IL-17RA and TRAF6 and so blocking the TRAF6-dependent pathway. To determine how IL-17A-induced signalling may be able to overcome this regulatory effect of IL-17RD, we examined the effect of IL-17A on the interaction of both IL-17RA and Act1 with overexpressed IL-17RD. Both IL-17RA and Act1 interacted basally with IL-17RD in unstimulated cells and these interactions were lost upon IL-17A stimulation ( Fig. 5d ). Interestingly, the time-dependent loss of binding of IL-17RD to IL-17RA and Act1, in response to IL-17A stimulation, closely correlates with IL-17A-induced binding of Act1 to IL-17RA and TRAF6 ( Fig. 5c ). These data suggest that IL-17RD may sequester Act1 and serve to prevent its interaction with IL-17RA and TRAF6. As IL-17RA, Act1 and IL-17RD have SEFIR domains, we next explored whether the SEFIR domain of IL-17RD was crucial for its interaction with Act1 and IL-17RA. An IL-17RD deletion mutant, termed IL-17RD ΔC, was generated that lacked the C-terminal SEFIR domain and was compared with its full-length counterpart for the ability to interact with Act1. Full-length IL-17RD interacted with coexpressed Act1 but IL-17RD ΔC failed to show any detectable interaction with Act1 ( Fig. 5e ). IL-17RD ΔC also failed to mimic full-length IL-17RD in its interaction with IL-17RA ( Supplementary Fig. S4 ), indicating an important role for the SEFIR domain of IL-17RD in facilitating interaction with IL-17RA and Act1. Furthermore, whereas overexpression of IL-17RD reduced the interaction of Act1 with TRAF6, IL-17RD ΔC had no effect on this interaction ( Fig. 5f ). These data are consistent with IL-17RD associating with IL-17RA and Act1 via a SEFIR–SEFIR interaction with this association being important for disrupting the Act1/TRAF6 signalling pathway. Indeed, this is further supported by full length IL-17RD inhibiting Act1-induced activation of NF-κB, whereas IL-17RD ΔC failed to show such inhibitory effects ( Fig. 5g ). Furthermore, IL-17RD was shown to have no effect on the TRAF6-independent mRNA stability pathway and indeed IL-17RD had no effect on the interaction of Act1 and IKKi ( Supplementary Fig. S5 ). These findings are consistent with a model where IL-17RD sequesters Act1 from interacting with IL-17RA and TRAF6 and so negatively regulates IL-17A-induced activation of NF-κB. Furthermore, stimulation of cells with IL-17A leads to dissociation of Act1 from IL-17RD and thereby allows interaction of the former with IL-17RA and TRAF6, thus triggering the NF-κB pathway. This provides a plausible mechanism by which IL-17RD can downregulate NF-κB-responsive genes such as IL-6 and KC . Interestingly, the sequestration of Act1 as a regulatory mechanism is not without precedent given that it can be targeted to prevents its inhibitory effects on B-cell activating factor receptor signalling [27] . Intriguingly, the earlier studies above also show that IL-17RD mediates IL-17A-induced expression of MIP-2 and neutrophilia and this appears at odds with a negative role for IL-17RD in IL-17 signalling. However, we demonstrated above that IL-17A-induced activation of the p38 MAPK pathway is dependent on IL-17RD and thus we assessed whether p38 MAPK mediates IL-17A-induced expression of MIP-2. IL-17A-induced activation of MIP-2 was abrogated in cells pretreated with the p38 MAPK inhibitor SB203580 ( Fig. 5h ). This is consistent with a previous report showing a requirement for p38 MAPK for MIP-2 expression in response to IL-17A [17] . Interestingly, the p38 MAPK inhibitor failed to affect KC expression and again this is consistent with the differential effect of IL-17RD on KC and MIP-2 expression. Although functional IL-17 cytokine signalling is associated with efficient clearance of extracellular pathogens, dysregulation of signalling can be damaging in exacerbating chronic inflammation and autoimmunity if not stringently regulated. The complexity of IL-17 biology is due to multiple members of the IL-17 family employing a number of IL-17 receptors with receptor co-operativity also being a feature of IL-17 action. On the basis of structural similarity the IL-17 receptor family is constituted by five members [28] . To date, direct functional data has demonstrated a role for only four of the IL-17 receptors (A, B, C and E) in IL-17 signalling. Despite sharing structural features with these other family members, IL-17RD remains an orphan receptor with no available data indicating a physiologically relevant role for IL-17RD in IL-17 biology. We now report for the first time, a regulatory role for IL-17RD in IL-17A-induced neutrophilia and activation of MAPK and NF-κB signalling pathways. Previous findings have demonstrated that IL-17RA, -B, -C and -E, but not IL-17RD, are upregulated upon IL-17A stimulation [7] . Instead basal IL-17RD expression is relatively high compared with IL-17RA and this is consistent with our proposed role for the orphan receptor acting as a basal 'braking system' that needs to be relieved by IL-17A stimulation in order to manifest the activation of NF-κB and induction of pro-inflammatory cytokines and chemokines. Importantly, IL-17RD appears to act to differentially regulate various IL-17-responsive genes. Although IL-17RD negatively regulates IL-17-induced expression of pro-inflammatory genes, such as IL-6 and KC , it also fulfils a key mediatory role in facilitating IL-17-induced expression of other pro-inflammatory proteins such as MIP-2. Indeed in an inflammatory context, the latter positive role of IL-17RD in IL-17 signalling appears to be the dominant one at least in the context of IL-17A-induced neutrophilia, as in the present study IL-17RD-deficient mice show greatly diminished neutrophil recruitment in tissues challenged with IL-17A. We also provide a mechanistic basis to the differential effects of IL-17RD on IL-17-responive genes. We propose that IL-17RD negatively regulates NF-κB by sequestering Act1 and preventing its interaction with IL-17RA and TRAF6, thus inhibiting ubiquitination of the latter. Sequestration of Act1 by IL-17RD is lost upon IL-17A stimulation, suggesting that IL-17RD inhibits Act1 function in resting cells and that this basal braking system is relieved upon stimulation of cells with IL-17 allowing for downstream activation of NF-κB and induction of genes such as IL-6 and KC . Intriguingly, IL-17RD also appears to have a contrasting mediatory role in IL-17A-induced phosphorylation of p38 MAPK and induction of MIP-2. The latter is especially important in terms of a critical physiological role for IL-17A in mediating tissue neutrophilia. Such findings also emphasize the complexity of the IL-17A signalling pathway. To date IL-17 signal transduction has been divided into TRAF6-dependent and TRAF6-independent pathways, the former assumed to trigger activation of NF-κB and MAPKs whereas the latter regulates mRNA stability. However, the present study clearly shows that IL-17RD can differentially regulate both the NF-κB and p38 MAPK pathways. Although IL-17RD negatively regulates TRAF6 ubiquitination and thereby inhibits NF-κB, it can also employ unubiquitinated TRAF6 to trigger activation of p38 MAPK. The exact mechanistic basis to these differential effects awaits full delineation. Previously, it has been reported that IL-17RD promotes IL-17A-induced signalling based on its ability to activate a 24p3 native promoter [23] . 24p3 or murine lipocalin-2 (also known as SIP24) is an IL-17-inducible gene that is dependent on NF-κB activation [29] . Such a positive role for IL-17RD in activation of a NF-κB-responsive promoter appears to directly contrast with our observed inhibitory function for IL-17RD in the NF-κB pathway. However, NF-κB recruitment to the 24p3 promoter has been reported to be dependent on p38 MAPK activity [30] and thus the presently described role for IL-17RD in mediating IL-17-induced activation of p38 MAPK may underlie the ability of IL-17RD to activate the 24p3 promoter [23] . Collectively, these data indicate that IL-17RD is an important functional regulator of IL-17A-induced signalling. Furthermore, IL-17RD is the last orphan receptor of the IL-17 receptor family and the present study prompts renewed interest in identification of a potential ligand for the IL-17RD receptor. This study reveals the first immunomodulatory and physiological role of IL-17RD and represents an important advance in our increasing awareness of the complexity of signalling triggered by IL-17 and its receptors. Mice IL-17RD-deficient mice were generated by the German Genetrap Consortium using its proprietary technology (Clone ID: D065E01) ( Supplementary Fig. S1a ). The genetrap targeting vector, which contains a promoter-less reporter gene downstream of a splice acceptor and a selectable marker gene ( β-Geo for β-Galactosidase neomycin-resistant fusion gene), was incorporated into the Il17rd gene after the first exon. The targeting vector contains loxP, f3 and lox5171 sites allowing conditional mutagenesis or recombinase-mediated cassette exchange. After the targeting vector was transfected into embryonic stem cells, G418-resistent colonies were selected and screened by PCR. Homologous recombinants were microinjected into female C57BL/6 background mice and heterozygous F1 progeny were intercrossed to obtain Il17rd −/− mice. Il17rd +/− mice were bred to generate age- and sex-matched Il17rd +/+ and Il17rd −/− mice for experiments. Breeding, colony expansion and maintenance were performed in the Bioresource facility of the National University of Ireland (NUI) Maynooth. All animals were housed in a barrier unit, in individually ventilated cages with high-efficiency particulate air filters. Animals are monitored regularly for microorganisms according to FELASA recommendations. All animal experiments were performed in accordance with the regulations and guidelines of the Irish Department of Health and protocols approved by the Research Ethics committee of NUI Maynooth. Plasmids and reagents Full-length IL-17RD was cloned from HEK293 cell cDNA. The primers for IL-17RD were designed based on the sequence deposited in GenBank (accession number AF458067 ). IL-17RD was tagged at the C-terminus with the c-Myc epitope tag by incorporating the c-Myc sequence in the reverse primer. Each forward and reverse primer contained Xba 1 restriction sites as underlined: forward 5′-GCTCTAGAGCATGGCCCCGTGGCTGCAGCTCTGCTCCGT-3′ and reverse 5′-GCTCTAGAGCTCACAGATCTTCTTCAGAAATAAGTTTTTGTTCCAAAGGGGCGACCGCGTGGAGTTC-3′. The PCR product was purified and subsequently cloned into the pcDNA3.1/Zeo (Invitrogen). IL-17RD ΔC was generated using the reverse primer 5′-GCTCTAGAGCTCACAGATCTTCTTCAGAAATAAGTTTTTGTTC ATAGCAGAGAA-3′. FLAG- and HA-tagged Act1 plasmids were gifts from Dr Antonio Leonardi (Federico II University of Naples, Italy). TRAF6 was from Tularik (San Francisco, CA) and IKKi was a gift from Dr Marion Butler (NUI, Maynooth, Ireland). TK Renilla -luciferase reporter construct (phRL-TK) was from Promega (Madison, WI). The NF-κB-luciferase reporter construct was a gift from Professor Luke O'Neill (Trinity College Dublin, Ireland). Tumour necrosis factor-α, IL-8 and β-actin 3′UTR luciferase constructs were gifts from Professor Andrew Bowie (Trinity College Dublin, Ireland). Recombinant mouse IL-17A was from R&D Systems (Minneapolis, USA) whereas recombinant mouse IL-17C, D, E and F were from ImmunoTools (GmbH, Friesoythe, Germany). Recombinant human IL-17A was from Peprotech (Rocky Hill, NJ, USA). Anti-phospho IκBα, anti-phospho IKK, anti-IKK, anti-phospho p38, anti-p38, anti-phospho ERK, anti-ERK, anti-phospho JNK, anti-JNK and anti-Myc antibodies were from Cell Signalling Technology Inc. (Danvers, MA). Anti-β-actin and anti-FLAG antibodies and Actinomycin D were supplied by Sigma-Aldrich. Anti-IκBα, anti-TRAF6, anti-ubiquitin, anti-Act1 and anti IL-17RA antibodies were from Santa Cruz Biotechnology (Santa Cruz, CA) and anti-HA antibody was from Covance Inc. (New Jersey, USA). Anti-CD11b, PE anti-Ly6G and APC anti-F4/80 antibodies were from eBioscience (San Diego, CA). p38 MAPK inhibitor SB203580 was from Calbiochem (Darmstadt, Germany). Cell Culture HeLa, HEK293 and U373 cells were cultured in Dulbecco's modified Eagle's medium supplemented with 10% (v/v) fetal bovine serum, 100 U ml −1 penicillin and 100 μg ml −1 streptomycin. Cells were maintained at 37 °C in a humidified atmosphere of 5% CO 2 . For the preparation of primary MEFs, Il17rd +/− mice were crossed to generate Il17rd +/+ and Il17rd −/− embryos. Embryos were dissected from pregnant females at day 13 post coitum. MEFs were isolated by standard procedure and cultured in Dulbecco's modified Eagle's medium supplemented with 10% (v/v) FBS for 3 days. To isolate marrow-derived macrophages, tibias and femurs from either Il17rd +/+ and Il17rd −/− mice were removed using sterile technique and the bone marrow was flushed with fresh medium. To obtain macrophages, cells were plated in medium supplemented with M-CSF (20 ng ml −1 ) and maintained at 37 °C in a humidified atmosphere of 5% CO 2 for 4–6 days. Human PBMCs from healthy volunteers were extracted from buffy coats provided by the Irish Blood Transfusion Service. PBMCs were isolated using the Ficoll-Hypaque isolation technique and plated in complete RPMI 1640 medium. Peritoneal and pulmonary administration of IL-17A Age- and sex-matched Il17rd +/+ and Il17rd −/− mice were treated with 0.5 μg of IL-17A (R&D Systems) by intraperitoneal injection, as previously described [31] , or 1 μg of the formyl–Met–Leu–Phe peptide (Sigma) prepared in endotoxin-free phosphate-buffered saline (PBS) and control mice were injected with endotoxin-free PBS. For the exogenous MIP-2 administration experiment mice were subjected to intraperitoneal injection of 0.5 μg of IL-17A or PBS 1 h before the treatment with recombinant murine MIP-2 (30 ng) for 2 h. The peritoneal cavity was lavaged with 2 ml ice-cold PBS at 0–6 h post treatment. Peritoneal cells were counted and quantified by flow cytometry and differential cell counting. To induce pulmonary neutrophilia, 0.5 μg IL-17A was introduced intranasally to groups of age-matched female Il17rd +/+ and Il17rd −/− mice as previously described [32] . After 4 h, bronchoalvelolar lavage (BAL) was performed and cellular infiltration into the lung was quantified by differential cell counts on BALs as previously described [33] . Lung tissue was perfused and fixed in 10% formalin saline. Paraffin-embedded sections were stained with hematoxylin and eosin to assess leukocyte infiltration and pulmonary inflammation. Lentiviral production and transduction HEK293T cells were seeded (2×10 5 cells ml −1 ; 3 ml) in six-well plates and grown for 24 h to~80% confluency. Cells were transfected using Lipofectamine 2000 (Invitrogen) according to the manufacturer's instructions with the packaging plasmid pCMV-dR 8.91 (1 μg), envelope plasmid VSV-G (1 μg) and IL-17RD sh-pLKO.1 vector (2 μg) or control shRNA (Sigma Aldrich, St. Louis, USA): IL-17RD shRNA 5′- CCGGCCAGTCTTGGAGAAATTTGATCTCGAGATCAAATTTCTCCAAGACTGGTTTTTG-3′ (NM_017563.1-1819s1c1). Conditioned medium was changed 24 h post transfection and replaced with fresh growth medium containing 30% (v/v) FBS for a further 24 h. The lentivirus-containing medium was harvested and replenished every 24 h for 72 h. U373 cells, seeded (2×10 5 cells ml −1 ; 3 ml) in six-well plates, were transduced with 600 μl lentivirus-containing medium with polybrene (8 μg ml −1 ) and incubated at 37 o C for 24 h before positive selection of cells with integrated shRNA constructs with puromycin (8 μg ml −1 ). Luciferase reporter assay HeLa and HEK293 cells were seeded (0.8×10 5 and 1.5×10 5 cells ml −1 , respectively) in 96-well plates (200 μl per well) for 24 h. Cells were then transfected using Lipofectamine 2000 (Invitrogen) according to the manufacturer's instruction, with luciferase reporter construct (80 ng), constitutively expressed TK Renilla -luciferase reporter construct (phRL-TK) (20 ng) (Promega Biosciences) and varying amounts of expression constructs. Total DNA was kept constant (200 ng per well) using the appropriate empty vector. For siRNA experiments, cells were transfected using Lipofectamine, with siRNA targeting IL-17RD (sense sequence: 5′-GGAGCAAACUACAGAGAUGTT-3′) or with scrambled siRNA (sense sequence: 5′-GGACAGAACACUAGAUGAGTT-3′) (10 nM and 20 nM) (Ambion). Cell extracts were generated 24 h (or 48 h for siRNA) post transfection using reporter lysis buffer (Promega Biosciences) and extracts were assayed for firefly luciferase and Renilla -luciferase activity using the luciferase assay system (Promega Biosciences) and coelenterazine (0.1 μg ml −1 Insight Biotechnology Ltd.), respectively. Luminescence was monitored with the Glomax microplate luminometer (Promega). Enzyme-linked immunosorbent assay MEFs or U373 cells, stably transfected with IL-17RD-specific shRNA or control shRNA, were seeded (3×10 5 cells ml −1 ; 200 μl) in 96-well plates and grown for 24 h. Cells were subsequently stimulated with various ligands for the indicated time points as described in figure legends. PBMCs were seeded (1×10 6 cells ml −1 ; 200 μl) in 96-well plates and after 2 h were transfected with siRNA (10 or 20 nM diluted in serum-free RPMI) using Lipofectamine 2000. An identical second transfection of siRNA with Lipofectamine 2000 was carried out 24 h later. After a further 24 h cells were stimulated with IL-17A (100 ng ml −1 ) for 24 h. Conditioned media from cells was measured for levels of murine IL-6, KC and MIP-2 or human IL-6, IL-8 and MIP-2 by sandwich enzyme-linked immunosorbent assay (ELISA; IL-6 and IL-8 DuoSet kits (R&D Systems), MIP-2 kits (Peprotech)). ELISA was also performed on lavage fluid from mice treated with PBS or IL-17A by intraperitoneal injection. Lavages were concentrated using Amicon-4 centrifugal filters (Millipore) before ELISA analysis. Electrophoretic mobility shift assay U373 cells, stably transduced with IL-17RD shRNA or control shRNA, and MEFs were grown in 90-mm dishes for 24 h. Cells were then stimulated with IL-17A (100 ng ml −1 ) for various times. Nuclear extracts were generated as previously described [34] . Nuclear protein (10 μg) was incubated with LI-COR IRDye 700 labelled oligonucleotide containing the NF-κB binding site 5′-AGTTGAGGGGACTTTCCCAGGC-3′ (κB site underlined), according to the manufacturer's instructions. For competitive analysis, unlabelled oligonucleotide was added to the extracts for 15 min before incubation with labelled oligonucleotide. All incubations were subjected to electrophoresis on a 4% native polyacrylamide gel for 2 h at 110 V and subsequently analysed and images captured using the Odyssey Infrared Imaging System (LI-COR Biosciences). Statistical analysis Data are expressed relative to untreated cells and are the means±s.e.m. of triplicate determinations from three independent experiments. For comparison between two groups, paired Student's t test (two tail, one type) was used. A P -value of <0.05 was considered significant. Genotyping of mice, co-immunoprecipitations, immunoblotting, RNA isolation, quantitative PCR, flow cytometry and slide preparation methodology are detailed in the Supplementary Method section. How to cite this article : Mellett, M. et al . Orphan receptor IL-17RD tunes IL-17A signalling and is required for neutrophilia. Nat. Commun. 3:1119 doi: 10.1038/ncomms2127 (2012).